Coordinated regulatory variation associated with gestational hyperglycaemia regulates expression of the novel hexokinaseHKDC1 Maternal glucose levels during pregnancy impact the developing fetus, affecting metabolic health both early and later on in life. Both genetic and environmental factors influence maternal metabolism, but little is known about the genetic mechanisms that alter glucose metabolism during pregnancy. Here, we report that haplotypes previously associated with gestational hyperglycaemia in the third trimester disrupt regulatory element activity and reduce expression of the nearby HKDC1 gene. We further find that experimentally reducing or increasing HKDC1 expression reduces or increases hexokinase activity, respectively, in multiple cellular models; in addition, purified HKDC1 protein has hexokinase activity in vitro . Together, these results suggest a novel mechanism of gestational glucose regulation in which the effects of genetic variants in multiple regulatory elements alter glucose homeostasis by coordinately reducing expression of the novel hexokinase HKDC1 . Regulation of glucose metabolism during pregnancy differs markedly from the non-gravid state as the mother must meet both her own and the growing fetus’s energy needs. The differences are characterized by the combination of lower fasting glucose levels, increased hepatic glucose output, increased nutrient-induced insulin secretion and significant insulin resistance by the third trimester [1] . In 5–10% of pregnancies, however, glucose homeostasis is not maintained, resulting in hyperglycaemia and gestational diabetes, that is, diabetes that is first diagnosed during pregnancy. Gestational hyperglycaemia is a major health risk to the mother, and is associated with adverse fetal outcomes including increased risk of type 2 diabetes and obesity in the offspring [2] , [3] , [4] , [5] . Despite the prevalence of health risks, the mechanisms leading to gestational hyperglycaemia remain largely unknown. We recently identified a strong association between genetic variants in the first intron of HKDC1 and 2-h plasma glucose levels during an oral glucose tolerance test performed in a multiethnic cohort of 4,437 mothers at ~28 weeks’ gestation (F-test, P =8.26 × 10 −13 , β =0.167–0.229 √[mmol l −1 ]; ref. 6 ). The association was replicated in a cohort of 2,192 additional European mothers and two smaller independent European and Canadian cohorts ( n =228 and 606). In a separate study of ~47,000 non-gravid individuals of European ancestry, the same region had only marginal association with 2-h plasma glucose, suggesting that the association with HKDC1 is largely pregnancy specific [7] . In the 1000 Genomes Project database (1KGP), there are 60 variants in the coding exons of HKDC1 . Seven of those variants are common, defined by a minor allele frequency >1%. According to computational predictions of the effects of those variants on HKDC1 activity, between one and four of the common variants may impact the function of HKDC1 (refs 8 , 9 ; Supplementary Data 1 ). However, none of the coding single-nucleotide polymorphisms (SNPs) were associated with 2-h plasma glucose at genome-wide significance ( P <1 × 10 −8 ). While the function of HKDC1 is unknown, the gene is broadly expressed including in liver and β-islet cells [6] , [10] ; conserved across vertebrates; and may be a novel human hexokinase based on its sequence similarity to hexokinase I ( HK1 ; ref. 11 ). On the basis of these data, we hypothesized that genetic variation that alters gene regulation may contribute to the association with gestational hyperglycaemia. Here we show that there are multiple variants that alter regulatory element activity in the region. Moreover, the effects of those variants are coordinated across four enhancer elements in the associated HKDC1 locus. For each variant, alleles associated with reduced expression also associate with higher plasma glucose in mothers. We further show that modulating HKDC1 levels alters hexokinase activity in multiple cellular models, and that purified HKDC1 protein has hexokinase properties in vitro. Together, our results support a novel mechanism of gestational glucose regulation in which coordinated variation across multiple enhancer elements within regulatory haplotypes reduces expression of the novel hexokinase HKDC1 . Identification of regulatory variants in the HKDC1 locus The strongest genetic association with 2-h plasma glucose was located within the first intron of HKDC1 at rs4746822. 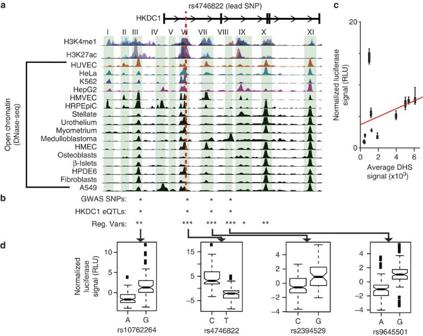Figure 1: Coordinated allelic regulation ofHKDC1. (a) Map of chromatin landscape and the HKDC1 genome-wide association (GWA) locus target regions. Evidence of active regulatory elements—genomic regions with the covalent histone modifications H3K4me1 and H3K27ac as measured by ChIP-seq and open chromatin measured by DNase-seq—is shown across the genomic locus associated with gestational hyperglycaemia. Green boxes indicate candidate the regulatory elements whose activity was measured with luciferase reporter assays. Histone modification and open chromatin data were obtained from the ENCODE project. (b) Coordinated regulatory variation in theHKDC1locus. SNPs that are significantly associated with gestational hyperglycaemia (‘GWA SNPs’),HKDC1mRNA expression (‘HKDC1 eQTLs’) or regulatory activity in allele-specific luciferase reporter assays (‘Reg. Vars’) are marked with an asterisk. (c) For each regulatory element ina, the enhancer activity (yaxis) is plotted against DNase-seq signal averaged across the element (xaxis) in HepG2 cells (n=8 to 19). Enhancer activity was determined by dividing the relative luciferase signal from the most active haplotype by that of a control vector with the same promoter but no enhancer. The red line indicates the Pearson correlation between DNase-seq signal and enhancer activity. Error bars show standard deviation (s.d.). (d) Example box plots showing allele-specific regulatory activity for the four SNPs that were significantly associated with gestational hyperglycaemia,HKDC1expression and luciferase reporter gene expression. In each example, allele associated with increased 2 h plasma glucose are shown in bold. The bottom and top boxes are the first and third quartiles, and the band inside the box is the median. The ends of the whiskers represent the lowest and highest data points within 1.5 interquartile range of the lower and upper quartiles. Black squares represent outliers defined as 1.5 × the interquartile range above the upper quartile or below the lower quartile. The number of replicate measurements followed by each allele are as follows: 103 of rs10762264A, 79 of rs10762264G, 80 of rs4746822C, 115 of rs4746822T, 129 of rs2394529C, 47 of rs2394529G, 80 of rs9645501A and 80 of rs9645501G. That variant and variants in moderate linkage disequilibrium (LD) with rs4746822 ( r 2 >0.3) lie within a region of the genome exhibiting chromatin modifications consistent with active gene regulation across diverse tissues ( Supplementary Figs 1 and 2 , Supplementary Table 1 ). To investigate the potential for regulatory variation contributing to the association with gestational hyperglycaemia, we focused on a ~30 kb region defined both by the observed pattern of LD in the region and by evidence of gene regulation. As shown in Supplementary Fig. 2 , there is little evidence of regulatory activity immediately flanking the target region, increasing our confidence that any regulatory variants contributing to the genetic association will be evaluated. There were three genotyped variants and nine imputed variants in the target region that were associated with 2-h plasma glucose at genome-wide significance ( P <1 × 10 −8 , Supplementary Data 2 ). Together, those data led us to hypothesize that rs4746822 or variants in LD with rs4746822 influence maternal glucose metabolism by altering the activity of regulatory elements that control HKDC1 expression. Within the target region, we identified 11 candidate regulatory elements on the basis of increased chromatin accessibility across 16 tissues including the metabolically relevant liver stellate cells and pancreatic islet β cells, ( Fig. 1a , Supplementary Table 1 ) [12] , [13] . The candidate regulatory regions account for 8.5 kb (28%) of the nucleotides in the 30 kb target region. Of the 425 variants in the target region identified by the 1KGP, 132 (30%) were in the candidate regulatory elements [14] . There were 203 total haplotypes of the individual regulatory elements, 60 of which were common in the 1KGP population (haplotype frequency >1%). 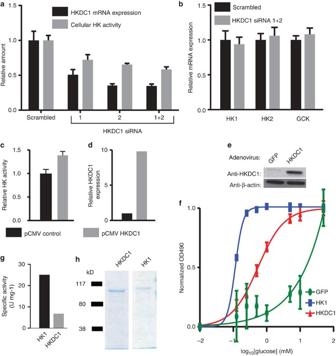Figure 2: HKDC1 is a hexokinase. (a) Two different siRNAs were used to knock downHKDC1in HepG2 cells. Quantification of hexokinase (HK) activity from whole-cell lysates shows a dose-dependent decrease in HK activity with reducedHKDC1expression (n=4). (b) siRNAs are specific toHKDC1and do not impact the expression of the other human hexokinase genes that are expression in HepG2 cells (n=4). (c,d) Transient overexpression ofHKDC1increases the total hexokinase activity in HepG2 cells compared with controls, which were transfected with a plasmid expressing a truncatedHKDC1mRNA (n=2). (e,f) Adenoviral-mediated overexpression of HKDC1 overexpression in INS-1 cells increased the amount of HKDC1 protein and cellular HK activity across a range of 0–50 mM glucose shown inf. The level of hexokinase activity was determined by dividing the optical density at 490 nm (OD490) at each glucose concentration by the OD490 at 50 mM glucose in all the three transduction conditions, respectively (n=3). (g) HKDC1 and HK1 protein was expressed in bacterial cells and isolated. Purity of the isolated protein was demonstrated with Coomassie blue staining. (h) Hexokinase assays performed on the purified protein demonstrate that both HKDC1 and HK1 have hexokinase activity. Specific activity was defined as micromoles of NADPH generated per hour per microgram of protein (n=2). All error bars in the figure show s.d. The 60 common haplotypes accounted for 98% haplotypes for the regulatory elements sequenced by the 1KGP ( Supplementary Table 2 ). Figure 1: Coordinated allelic regulation of HKDC1. ( a ) Map of chromatin landscape and the HKDC1 genome-wide association (GWA) locus target regions. Evidence of active regulatory elements—genomic regions with the covalent histone modifications H3K4me1 and H3K27ac as measured by ChIP-seq and open chromatin measured by DNase-seq—is shown across the genomic locus associated with gestational hyperglycaemia. Green boxes indicate candidate the regulatory elements whose activity was measured with luciferase reporter assays. Histone modification and open chromatin data were obtained from the ENCODE project. ( b ) Coordinated regulatory variation in the HKDC1 locus. SNPs that are significantly associated with gestational hyperglycaemia (‘GWA SNPs’), HKDC1 mRNA expression (‘HKDC1 eQTLs’) or regulatory activity in allele-specific luciferase reporter assays (‘Reg. Vars’) are marked with an asterisk. ( c ) For each regulatory element in a , the enhancer activity ( y axis) is plotted against DNase-seq signal averaged across the element ( x axis) in HepG2 cells ( n =8 to 19). Enhancer activity was determined by dividing the relative luciferase signal from the most active haplotype by that of a control vector with the same promoter but no enhancer. The red line indicates the Pearson correlation between DNase-seq signal and enhancer activity. Error bars show standard deviation (s.d.). ( d ) Example box plots showing allele-specific regulatory activity for the four SNPs that were significantly associated with gestational hyperglycaemia, HKDC1 expression and luciferase reporter gene expression. In each example, allele associated with increased 2 h plasma glucose are shown in bold. The bottom and top boxes are the first and third quartiles, and the band inside the box is the median. The ends of the whiskers represent the lowest and highest data points within 1.5 interquartile range of the lower and upper quartiles. Black squares represent outliers defined as 1.5 × the interquartile range above the upper quartile or below the lower quartile. The number of replicate measurements followed by each allele are as follows: 103 of rs10762264A, 79 of rs10762264G, 80 of rs4746822C, 115 of rs4746822T, 129 of rs2394529C, 47 of rs2394529G, 80 of rs9645501A and 80 of rs9645501G. Full size image To determine whether genetic variation in the identified regulatory elements influences endogenous HKDC1 expression, we compared the variants associated with gestational hyperglycaemia to those associated with gene expression changes in an expression quantitative trait locus (eQTL) study performed in primary human livers [15] . To do so, we imputed the tag variants from both the GWA and eQTL studies to the variants identified in the 1KGP [14] . That analysis revealed four significant eQTLs for HKDC1 [log 10 (Bayes Factor)>2.5] within DNaseI hypersensitive sites (DHS) that were also associated with maternal 2-h glucose levels ( Fig. 1b , Supplementary Fig. 2 , Supplementary Data 3 ). We did not find evidence that the same variants also influence expression of nearby HK1 in the same study ( Supplementary Data 4 ), and known HK1 eQTLs in other cell types do not overlap the variants associated with maternal glucose levels [16] . When we expanded our eQTL analysis to all genes within 500 kb of HKDC1 , we did not find any evidence that variants associated with 2-h maternal glucose levels were also eQTLs for those genes ( Supplementary Fig. 3 ). Together, these results suggest that genetic variants associated with gestational hyperglycaemia near HKDC1 alter HKDC1 expression. To identify causal variants that control HKDC1 expression, we used luciferase reporter assays to measure allele-specific regulatory activity of the candidate regulatory elements in the region in the HepG2 liver cell line. We identified 1KGP subjects that maximized the genetic diversity in the candidate regulatory elements, and used PCR to clone the regulatory elements from those individuals upstream of a Simian Virus 40 promoter driving expression of a luciferase reporter gene. From the genomes of 19 individuals ( Supplementary Table 3 ), we cloned 60 different naturally occurring haplotypes representing 93% of the haplotypes of the 11 regulatory elements that were identified by the 1KGP. To disentangle the effects of individual variants that do not segregate in the population on expression and to increase our power to detect regulatory effects of variants that are rare in the population, we used site-directed mutagenesis to generate reporter constructs for 45 additional haplotypes ( Supplementary Data 5 ). By balancing the number of observations of each allele, we were able to alleviate some of the loss in power due to allele frequency differences ( Supplementary Table 4 ). In total, we assayed 105 haplotypes composed of 57 variants. Nine of the 11 regulatory elements had enhancer activity, with relative luciferase expression between 1.9- to 14-fold over control ( Supplementary Fig. 4 ). Enhancer strength was positively and significantly correlated with average DHS peak intensity in HepG2 cells (Spearman ρ =0.64, P <0.05, Fig. 1c ), however, we did not find significant correlation between DHS peak width and enhancer strength ( Supplementary Fig. 5 ). We do not take these results as evidence that DHS peak intensity generally predicts enhancer strength, only that DHS sites are enriched for active regulatory elements. To identify individual genetic variants in the regions that altered enhancer activity, we used a multiple linear regression model to estimate the effect of each variant acting independently on reporter expression ( Supplementary Data 6 , Supplementary Fig. 6 ). That analysis revealed 14 variants distributed across six regulatory elements that significantly altered gene expression (Bonferroni-adjusted P <0.01, Fig. 1b , Table 1 , and Supplementary Table 5 ). In agreement with other studies, we found that the effect of a single variant on enhancer activity is generally <2-fold [17] , [18] , [19] . We next determined if the estimated effects of individual variants within an element behaved cumulatively. For each of the six elements containing regulatory variants, we quantified the expected luciferase values for each haplotype by adding the coefficients on the basis of each variant within the haplotype and plotted those against the observed luciferase values. In all the six elements, predicted luciferase values were positively and significantly correlated with observed luciferase values (Pearson r 2 >0.25, P <0.0001, Supplementary Fig. 7 ). Although we observe substantial cumulative effects, we cannot dismiss the possibility that more complex interactions also exist. Table 1 Association of functional genetic variants with regulatory activity ( β -luciferase ( β -luc), HKDC1 expression ( β -eQTL) and gestational hyperglycaemia ( β -GWA). Full size table The results from the allele-specific reporter assays were positively validated in the liver eQTL study. For 10 out of 12 variants present in the eQTL analysis, the effect observed in our allele-specific reporter assays was in the same direction as predicted by the eQTL association ( P =0.02, binomial test). Among the validated regulatory variants were four genome-wide significant eQTLs ( Fig. 1d , Table 1 ). The observed effects of those four variants in our reporter assays were not specific to HepG2 cells. Specifically, in seven of the eight cases in which one of the variants significantly altered regulatory element activity in a different cell type, the direction of the effect was consistent with that observed in HepG2 cells ( Supplementary Table 6 ). Together, these results indicate that rs10762264, rs4746822, rs2394529 and rs9645501 are regulatory variants in four separate enhancers that contribute to HKDC1 expression in human liver. The identified regulatory variants have coordinated effects For the regulatory variants identified to collectively contribute to maternal glycaemia, we hypothesized that there would be coordination between allele-specific regulatory element activity and maternal 2-h glucose levels. Supporting our hypothesis, all four variants that were significant eQTLs for HKDC1 in liver were associated with maternal 2-h glucose levels with three reaching genome-wide significance in the imputed GWA data ( Table 1 ). All four alleles that were associated with increased 2-h glucose also had decreased luciferase expression in the reporter assays and decreased HKDC1 expression in the eQTL analysis ( Fig. 1d , Table 1 ). We expanded the analysis to include 12 genome-wide significant SNPs associated with 2-h glucose and found that each of the 12 SNPs associated with increased glucose also associated with decreased HKDC1 expression ( P =0.0002, binomial test, Supplementary Data 7 ). We further expanded the analysis to include all 178 tested SNPs within the 30 kb locus and found the risk allele to decrease HKDC1 expression in 131 cases ( P =1.14 × 10 −10 , binomial test, Supplementary Data 7 ). Together, those results support a model in which multiple genetically linked regulatory variants have a coordinated effect of reducing HKDC1 expression in women with higher gestational glucose levels. Exceptions to the coordination were limited to variants that were not significantly associated with 2-h plasma glucose levels or HKDC1 expression and that were not in strong LD with the lead GWA variant. For rs7089277, the minor allele frequency is low (7%) and therefore the variant may have limited effects in the population, and there is only nominal association with 2-h glucose ( P =8.02 × 10 −5 ). The two SNPs in region X have large luciferase βs, but were not significantly associated with 2-h glucose ( P =0.0183 and 0.0184), were not in LD with rs4746822 ( r 2 =0.077) and did not significantly associate with HKDC1 expression. Furthermore, reporter assays in three additional cell types found cell-dependent effects for the variants in region X ( Supplementary Table 7 ). Together, these results indicate that there are strongly coordinated regulatory effects across the genomic region associated with 2-h plasma glucose levels, and that exceptions to that coordination likely do not contribute to the expression of HKDC1 . HKDC1 is a novel human hexokinase gene Having demonstrated that alleles associated with higher maternal 2-h glucose levels decrease HKDC1 expression, we next sought to understand whether HKDC1 has hexokinase activity that may explain its contribution to glucose homeostasis. Phosphorylation of glucose by hexokinase is the first step in glucose metabolism. Screens for hexokinase activity in rat cells have identified four distinct hexokinases using electrophoresis and chromatography. Those genes have been mapped, and are known as HK1 , HK2 , HK3 and glucokinase ( GCK ) [20] , [21] , [22] . Reduced hexokinase activity has previously been associated with metabolic phenotypes including diabetes [23] , [24] . To determine whether HKDC1 contributes to cellular hexokinase activity, we first used siRNA-mediated knockdown to model the genetically reduced levels of HKDC1 expression present in women with higher 2-h glucose concentrations, and measured the effect of that reduction on cellular hexokinase activity. Targeting HKDC1 with two different siRNAs individually and together in HepG2 cells, we reduced mRNA expression by 35–60%. Reduced HKDC1 expression resulted in a dose-dependent decrease in cellular hexokinase activity ( Fig. 2a ). The siRNAs were specific and did not alter expression of HK1 , HK2 or GCK ( Fig. 2b ). HK3 expression was not detectable in HepG2 cells, as expected [12] . The magnitude of reduction in hexokinase activity indicates that about half of the hexokinase activity in HepG2 cells is due to HKDC1 . That result agrees with RNA-seq data showing that half of the hexokinase mRNA expression in HepG2 cells is HKDC1 ( Supplementary Table 8 ). Providing further evidence that HKDC1 contributes to cellular hexokinase activity, we also found that overexpression of HKDC1 mRNA by transient transfection of an HKDC1 expression plasmid increased cellular hexokinase activity ( Fig. 2c,d ). Figure 2: HKDC1 is a hexokinase. ( a ) Two different siRNAs were used to knock down HKDC1 in HepG2 cells. Quantification of hexokinase (HK) activity from whole-cell lysates shows a dose-dependent decrease in HK activity with reduced HKDC1 expression ( n =4). ( b ) siRNAs are specific to HKDC1 and do not impact the expression of the other human hexokinase genes that are expression in HepG2 cells ( n =4). ( c , d ) Transient overexpression of HKDC1 increases the total hexokinase activity in HepG2 cells compared with controls, which were transfected with a plasmid expressing a truncated HKDC1 mRNA ( n =2). ( e , f ) Adenoviral-mediated overexpression of HKDC1 overexpression in INS-1 cells increased the amount of HKDC1 protein and cellular HK activity across a range of 0–50 mM glucose shown in f . The level of hexokinase activity was determined by dividing the optical density at 490 nm (OD490) at each glucose concentration by the OD490 at 50 mM glucose in all the three transduction conditions, respectively ( n =3). ( g ) HKDC1 and HK1 protein was expressed in bacterial cells and isolated. Purity of the isolated protein was demonstrated with Coomassie blue staining. ( h ) Hexokinase assays performed on the purified protein demonstrate that both HKDC1 and HK1 have hexokinase activity. Specific activity was defined as micromoles of NADPH generated per hour per microgram of protein ( n =2). All error bars in the figure show s.d. Full size image To demonstrate that the activity of HKDC1 was not specific to HepG2 cells, we transduced the rat pancreatic β-cell line, INS-1, with an adenovirus that expressed HKDC1 from a human cytomegalovirus promoter and measured hexokinase activity in the cell lysates at glucose concentrations ranging from 0 to 50 mM (ref. 25 ). The predominant hexokinase in INS-1 cells is GCK, and the cells have little or no detectable low K m hexokinase activity [25] . Cells transduced with the HKDC1 adenovirus had substantially increased HKDC1 protein ( Fig. 2e , Supplementary Fig. 8 ), and increased hexokinase activity across the concentration range ( Fig. 2f , Supplementary Fig. 9 ). Moreover, the shift in the dose–response curve suggests that HKDC1 has a lower K m than GCK. Adenoviral-mediated HKDC1 overexpression did not alter the expression of HK2 , HK3 or GCK and decreased HK1 , demonstrating that the virus specifically overexpressed HKDC1 ( Supplementary Fig. 10 ). Transduction also did not result in decreased cell density ( Supplementary Fig. 11 ). We repeated the experiment with independently purified virus and independently grown INS-1 cells, with similar results ( Supplementary Fig. 12 ). Together, these results demonstrate that HKDC1 contributes to cellular hexokinase activity either through direct hexokinase activity or through modulating the activity of the other hexokinases. On the basis of the extent of nucleotide and amino-acid similarity between HKDC1 and members of the hexokinase family, ( Supplementary Data 8 and 9 , Supplementary Tables 9 and 10 ), we hypothesized that the effects of HKDC1 expression on cellular hexokinase activity are in part the result of the direct enzymatic activity of HKDC1. To test that hypothesis, we purified HKDC1 and compared its specific activity to that of purified HK1. Protein purity was confirmed via a Coomassie blue stain ( Fig. 2g , Supplementary Fig. 8 ). Results of the assays indicate that HKDC1 protein alone has hexokinase activity, with 20% of the specific activity of HK1 under the same conditions ( Fig. 2h ). Because our results show HKDC1 hexokinase activity in vitro and in vivo , we propose renaming the HKDC1 gene to HK5 . We have shown that regulatory variation associated with gestational glucose metabolism alters expression of a novel human hexokinase. This result adds to the growing empirical evidence that regulatory variants contribute to a variety of common complex human phenotypes [26] , [27] , [28] . Moreover, our results provide empirical evidence that regulatory variants spanning multiple enhancers have a coordinated allelic effect on HKDC1 expression. A recent analysis suggests that such coordinated effects may be a common mechanism by which regulatory variants influence gene expression [26] . Such coordinated disruption of regulatory haplotypes may also explain how modest effects of individual regulatory variants [17] can together have a sufficiently strong effect so as to be detectable in a genome-wide genetic analysis. The burden of multiple genetic variants disrupting regulatory haplotypes may therefore help explain the overabundance of noncoding genetic variants in GWA studies. Notably, however, independent effects were not observed in our analysis of the liver eQTL data. This negative result may be explained by differences in effect size, limited power between closely linked variants and tissue-specific effects ( Supplementary Fig. 13 ). Together, we take the results presented here to be consistent with a model of coordinated regulatory variation, and we emphasize the need for additional investigation. In part, challenges of a strong association between variants and heterogeneous effect sizes may be overcome with high-throughput empirical investigation of allele-specific regulatory activity in large populations [17] , [29] . Importantly, the plasmid-based reporter assays used to detect regulatory variants here are likely biased towards detecting regulatory elements that act independent of genome context. Additional elements may be active when in the native genomic context, where interactions between multiple clustered regulatory elements contribute to effects on nearby gene regulation. Similarly, determining the direct effects variants detected here on endogenous gene expression remains a challenge. Addressing that possibility will require additional studies that include genomic context, potentially through direct modification of the genome via genome editing [30] , [31] . Studying regulatory effects in the locus associated with maternal glycaemia also led us to the discovery of a novel human hexokinase that appears to have important metabolic effects during pregnancy. Previous screens to identify vertebrate hexokinases [32] , [33] have identified HK1, HK2, HK3 and GCK, but did not identify HKDC1. One possible reason why HKDC1 was missed previously is that a high degree of structural similarity between HKDC1 and HK1 may have obscured separation in chromatography and electrophoresis. We also found that purified HKDC1 has reduced hexokinase activity when compared with HK1 in our in vitro assays. One possibility is that additional co-factors could be required for full HKDC1 activity in vitro , but that those factors are lost during the purification process. Such diminished hexokinase activity may have prevented earlier detection of HKDC1 as a hexokinase by less-sensitive methods. The tissues that are most relevant for the role of HKDC1 in meeting the metabolic demands of pregnancy are not yet known, nor is it known how HKDC1 is regulated in response to pregnancy hormones. We expect that future evaluation of these questions will provide new insights into the metabolic changes that occur during pregnancy. More broadly, the results from this study demonstrate the value of identifying and pursuing the targets of noncoding phenotype-associated genetic variants for revealing novel mechanisms of human disease [34] . Luciferase reporter assays The selected regions were amplified from genomic DNA from 1KGP subjects and In-Phusion cloned at the NheI cut site into pGL4.13 luciferase expression vector (Promega). The construct was then transformed into TOP-10 competent cells and plated onto Luria-Bertani agar plates with ampicillin and incubated overnight at 37 °C. In order to capture both haplotypes from subjects who were heterozygous in those regions, multiple colonies were selected and grown individually in Luri-Bertani media overnight. Plasmids were extracted using the PureYield Plasmid Miniprep System (Promega). Constructs were sequenced using Sanger sequencing and variants were confirmed in dbSNP [35] . Site-directed mutagenesis was carried out by amplifying the plasmid using primers containing the allele of choice, treating with DpnI and transforming into TOP-10 competent cells. Primers for cloning and site-directed mutagenesis are listed in Supplementary Tables 11 and 12 . HepG2 cells (Duke Cell Culture Facility)were plated into white flat-bottom 96-well plates at a density of 25,000 cells per well. After 48 h, 100 ng of each construct per well was transfected with Fugene HD (Promega) at a 5.5:1 Fugene:DNA ratio. At least 16 biological replicates for each construct were transfected. After 24 h, luciferase and renilla luciferase signal were quantified using the Dual-glo Luciferase Assay (Promega) using a Victor3 1420 plate reader (PerkinElmer). Luciferase values were normalized by dividing the luciferase signal by the renilla signal. A linear regression model implemented in the R statistical package (R function lm) was used to determine the regulatory effect of individual SNPs where (normalized luciferase intensity)=β 1 SNP 1 +β 2 SNP 2 +β 3 SNP 3 …+ ε. Raw data for luciferase reporter assays are provided as Supplementary Data Sets . Quantitative PCR with reverse transcription RNA was isolated using the RNeasy kit (Qiagen). Two micrograms of RNA per reaction was reverse transcribed using the SuperScript Vilo cDNA Kit (Life Technologies). All quantitative PCR (qPCR) reactions were performed in biological triplicates and technical duplicate using the PerfeCTa qPCR Fastmix (Quanta) on an ABI StepOnePlus cycler. Reactions were cycled at 95 °C (10 s) and the primer annealing temperature (30 s) for 40 cycles. Calculations were performed using the ΔΔC t method using β-actin as a reference control. Primer sequences are listed in Supplementary Table 13 . Western blots Transduced cell pellets were sonicated for 5 × 30 s pulses in 100 μl of RIPA buffer supplemented with protease inhibitors. The protein concentrations were quantified using a bicinchoninic acid assay (Thermo Scientific). The lysate was then mixed 1:1 with loading buffer supplemented with 5% 2-mercaptoethanol and incubated at 76 °C for 15 min. Then, 10 μg of protein along with the Precision Plus Protein Dual Color Standard (Bio-Rad) was loaded into each lane of a Mini-Protean TGX 4–20% gel (Bio-Rad) and run at 100 V for 1 h at 4 °C. The membrane was blocked with 5% skimmed milk for 30 min and washed three times in 0.1% Tween-20 in phosphate-buffered saline. The membrane was incubated overnight in anti-HKDC1 antibody produced in rabbit (Sigma) diluted 1:500 in skimmed milk. The membrane was washed three more times and incubated in horseradish peroxidase conjugated anti-rabbit antibody diluted 1:2,500 in skimmed milk for 75 min at room temperature (Santa Cruz Biotechnology). The membrane was washed three times and incubated at room temperature in 10 μl SuperSignal West Pico Chemiluminescent Substrate (Thermo Scientific) for 15 min. After exposure and imaging, the membrane was stripped using Restore Western Blot Stripping Buffer (Thermo Scientific) and blotted using 1:500 anti β-actin antibody produced in mouse (Santa Cruz Biotechnology) and 1:2,500 horseradish peroxidase conjugated anti-goat antibody (Santa Cruz Biotechnology) diluted in skimmed milk. Adenovirus construction and transduction A 2,789 bp BamHI/NotI fragment from plasmid RC221178 (OriGene), containing the 2,750 bp HKDC1 open reading frame, was cloned into the BamHI/NotI sites of the adenoviral shuttle vector pShuttle-CMV (Agilent). HKDC1 adenoviral shuttles were linearized with PmeI and transformed into BJ5183-AD1 cells (Agilent). Recombinant clones were isolated, digested with PacI and recombinant adenoviruses were generated by transfecting HEK293 cells (Clontech) with the PacI digested recombinant plasmid DNA and FuGene [36] . To generate the HK1 adenovirus, a 3,600 bp DNA fragment containing the rat HK1 ORF was cloned into the shuttle vector pAC.CMV.pLpA. Recombinant HKI virus was then generated by co-transfecting HEK293 cells with HKI shuttle clone and plasmid pJM17 (ref. 25 ). After transfection, viral lysate was collected, further amplified in HEK293 cells plated in 5 × p150 tissue culture plates. Before complete lysis, media was removed, infected cells collected in 2 ml freeze/thaw buffer (10 mM Tris/HCl, pH 8.0, 1 mM MgCl 2 ), lysed by two freeze/thaw cycles and the virus purified by ultracentrifugation on a CsCl gradient. Purified virus was de-salted with a 7k MWCO column (Thermo Scientific) equilibrated with freeze/thaw buffer, and glycerol was added to a final concentration of 10%. Viruses were titred by measuring OD 260 (1 OD 260 =1.1 × 10 12 virions ml −1 ) as well as by plaque assay in HEK293 cells. To prepare cells for transduction, INS-1 cells were first seeded at a density of 7 × 10 5 per well into 12-well plates. INS-1 832/13 cells were kindly provided by Christopher Newgard (DMPI, Duke University) [37] . After 24 h, the cells were transduced with HKDC1 -, HK1 - or GFP -expressing adenovirus in triplicate. Cells were grown for another 24 h and pelleted with centrifugation. Protein purification Rosetta 2 (DE3) (EMD Millipore) cells were transformed with pReceiver-B01 plasmid containing either HKDC1 or HK1 . A single colony was grown overnight in 100 ml TPM media (20 g l −1 Tryptone, 15 g l −1 yeast extract, 8 g l −1 NaCl, 2 g l −1 Na 2 HPO 4 1 g l −1 KH 2 PO 4 ) augmented with 50 μg ml −1 ampicillin and 34 μg μl −1 chloramphenicol at 37 °C. The pregrowth culture was added to 500 ml of the same media and grown to an OD of ~0.6. Isopropyl β- D -1-thiogalactopyranoside was added to a final concentration of 1 mM, and the cells were grown for an additional 4 h at room temperature. Cultures were centrifuged at 10,000 g for 30 m and resuspended in lysis buffer (50 mM NaH 2 PO 4 , 300 mM NaCl, 0.25% Tween-20, 5% sucrose, 5% glycerol, 2 mM imidazole and 10 mM 2-mercaptoethanol) supplemented with protease inhibitors (1 mM phenylmethanesulfonyl fluoride, 2 μg ml −1 aprotinin, 0.5 μg ml −1 leupeptin, 0.7 μg ml −1 pepstatin A). Cells were sonicated for 5 min followed by DNase I treatment (4 U ml −1 ) for 15 min on ice. The lysates were clarified by centrifugation at 10,000 g for 30 min and the supernatant passed over a HisTALON column (Clontech). The column was washed with 25 ml of wash buffer (Lysis buffer pH 7.0, 25 mM imidazole). The protein was eluted from the column in 1 ml fractions using wash buffer with 500 mM imidazole. DTT was added to each fraction to a final concentration of 1 mM. Cellular hexokinase assays To measure cellular hexokinase activity in knockdown and overexpression experiments, we used an absorbance-based hexokinase assay (Sciencell #8408). Cell pellets were sonicated in 200 μl of 1% Triton at 4 °C for 5 × 30 s pulses at medium intensity using a Bioruptor (Diagenode). The lysate was centrifuged at 1,000 g for 5 min to remove remaining cell debris. The assay was performed by combining 80 μl of reaction mix (42 μl assay buffer, 20 μl cofactor, 2 μl developer, 6 μl enzyme mix and 10 μl NADP), 10 μl of cell lysate and 10 μl of 0–500 mM glucose in each well of clear 96-well microplates. The plates were incubated in the dark for 90 min at room temperature. Absorbance at 490 nm was quantified in technical duplicates using a Victor3 1420 plate reader (PerkinElmer). Purified HKDC1 hexokinase assays To assay hexokinase (HK) activity of purified HKDC1, 2 μg of purified protein was diluted in 20 μl of HK dilution buffer containing 20 mM KH 2 PO 4 , 100 mM KCl, 1 mM MgCl 2 , 1 mM EDTA, 1 mM dithiothreitol (DTT), 60 g l −1 glycerol and 1 g l −1 bovine serum albumin. Samples were loaded onto a microplate and mixed with 100 μl of reaction buffer containing 50 mM HEPES pH 7.4, 100 mM KCl, 8 mM MgCl 2 , 5 mM ATP, 0.5 mM NADP, 1 U ml −1 G6PDH (from Leuconostoc mesenteroides ), 1 mM DTT, 1 g l −1 bovine serum albumin and 10 mM D -(+)-glucose. Reactions were incubated at 37 °C for 1 h and stopped with 174 μl buffer C (0.46 mM SDS pH 8.0, 300 mM NaH 2 PO 4 , pH 8.0). Fluorescence of NADPH was measured at excitation wavelength of 340 nm and an emission wavelength of 450 nm. Specific activity was determined using an NADPH standard ( Supplementary Fig. 14 ). Multiple sequence alignment Multiple sequence alignments and percent identity matrices were constructed using Clustal Omega using default settings http://www.ebi.ac.uk/Tools/msa/clustalo/ ) [38] . Protein and DNA sequences were downloaded from UCSC genome browser [39] . siRNA knockdown HepG2 cells were plated at 1 × 10 5 cells per well into 24-well plates. After 48 h, cells were transfected with either siRNAs targeting HKDC1 (Ambion Silencer Select s37044, s37046) or siRNA not known to target any genes (Ambion Silencer AM4611) using 6 pM of siRNA and 1 μl of Lipofectamine RNAiMax transfection reagent (Life Technologies) per well. Each siRNA was transfected in biological triplicate. Cells were collected 24 h later for RT–qPCR and hexokinase assays as described above. Genome-wide association with imputed genotypes Genotypes from the previously published GWA study that identified the HKDC1 locus [6] were imputed separately in each of the four quality control cleaned and filtered genotyping sets using IMPUTE2 v2.3.0 and the 1KGP reference panel (December 2013 release). A cosmopolitan reference panel of unrelated individuals of the African (‘AFR’), American (‘AMR’), Asian (‘ASN’) and European (‘EUR’) populations was used. The strand-checking utility of SHAPEIT v2 was used to ensure consistent strand assignments between the reference data set and the quality control cleaned and filtered data sets. Strand was corrected as indicated, and SNPs for which strand could not be resolved were removed. A conservative info threshold (synonymous to allelic r 2 ) of 0.9 was used to remove questionable imputed SNPs. The genotype call probabilities from the filtered IMPUTE2 output were used in a linear regression model between each of the phenotypes and the genotypes probabilities under an additive model adjusting for age, BMI and the first two principal components (PCs) of ancestry. The frequentist approach in SNPTEST v2.4.1 was used to estimate the beta and standard errors for each regression model and assess the significance of the association between the SNP and the phenotype of interest. Liver eQTL analyses Liver gene expression and genotype data were generated as follows [15] . Gene expression array probes were aligned to the human reference genome (hg19) and gene models (RefSeq). Probes lacking unique genomic or transcriptomic alignments were discarded. Furthermore, probes overlapping common polymorphisms (minor allele frequency >5%, based on 1KGP pilot release data) were discarded. Gene expression array feature intensities were extracted from arrays, background subtracted and log 2 transformed. Missing data were imputed by k nearest neighbours (R package impute, function impute.knn, k =10). The distribution of expression measurements on each array was normalized to the average empirical distribution across all arrays (R package limma, function normalizeBetweenArrays, method quantile). For each probe and across arrays, the distribution of expression values was transformed to the quantiles of the standard normal distribution (R function qqnorm). This matrix of processed gene expression values was then subjected to PCA (R package pcaMethods, function pca). We controlled for the effect of these PCs by taking the residuals of linear models using the first 15 PCs as covariates. Values from replicate arrays were then averaged. Because this sample set included both European and African American individuals, residual expression values were then transformed to the quantiles of the standard normal distribution within each population and then pooled. Given the mappings of probes to gene models, if there were multiple probes that mapped to the same gene, probes were clustered [R package mclust, function Mclust(y,G=1:min(4,probe_count))] and the mean per cluster per individual was estimated. These residuals were then transformed by gene to standard normal. These data were used as phenotypes for the eQTL scan. Genotype data were processed and quality controlled as follows [15] . Genotyping was performed on the Illumina human 610 quad beadchip platform (GPL8887) at the Northwestern University Center for Genetic Medicine Genomics Core Facility according to the manufacturer’s instructions. One sample was removed because it had a no-call rate >10%. The initial marker set comprised 620,901 markers. A total of 8,300 markers were removed because they showed significant deviation from Hardy–Weinberg equilibrium (Fischer’s exact test, P <0.001). A total of 29,705 SNPs were removed from the analysis because they had a no-call rate in >10% of the samples. Hence, our final marker set comprised 583,073 SNPs. Imputation was performed using impute2 and the full 1KGP reference panel, as per impute2 recommendations, in 5 Mb segments using the commands: impute_v2.2.2_x86_64_dynamic/impute2 -prephase_g -Ne 20000 impute_v2.2.2_x86_64_dynamic/impute2 -Ne 20000 The cis-eQTL scan was conducted with Bayesian regression using all SNPs within 1 Mb of the gene using the command: snptest_v2.5-beta4 -use_raw_phenotypes -bayesian 1 -method expected -pheno pheno1 -prior_qt_mean_b 0 -prior_qt_V_b 0.02 -prior_qt_a 3 -prior_qt_b 2 How to cite this article: Guo, C. et al . Coordinated regulatory variation associated with gestational hyperglycaemia regulates expression of the novel hexokinase HKDC1 . Nat. Commun. 6:6069 doi: 10.1038/ncomms7069 (2015).